Gut microbiome of the Hadza hunter-gatherers Human gut microbiota directly influences health and provides an extra means of adaptive potential to different lifestyles. To explore variation in gut microbiota and to understand how these bacteria may have co-evolved with humans, here we investigate the phylogenetic diversity and metabolite production of the gut microbiota from a community of human hunter-gatherers, the Hadza of Tanzania. We show that the Hadza have higher levels of microbial richness and biodiversity than Italian urban controls. Further comparisons with two rural farming African groups illustrate other features unique to Hadza that can be linked to a foraging lifestyle. These include absence of Bifidobacterium and differences in microbial composition between the sexes that probably reflect sexual division of labour. Furthermore, enrichment in Prevotella , Treponema and unclassified Bacteroidetes , as well as a peculiar arrangement of Clostridiales taxa, may enhance the Hadza’s ability to digest and extract valuable nutrition from fibrous plant foods. The human gut microbiota (GM) is vital for host nutrition, metabolism, pathogen resistance and immune function [1] , and varies with diet, lifestyle and environment [2] , [3] , [4] . Together, the host and microbiome have been termed a ‘supra-organism’ whose combined activities represent both a shared target for natural selection and a driver of adaptive responses [5] . By studying GM variation across human populations, we are able to explore the limits of our genetic and metabolic potential, and the extent to which GM-host co-evolution is responsible for our physiological flexibility and environmental adaptation [6] , [7] , [8] . Comparative studies between unindustrialized rural communities from Africa and South America and industrialized western communities from Europe and North America have revealed specific GM adaptations to their respective lifestyles. These adaptations include higher biodiversity and enrichment of Bacteroidetes and Actinobacteria in rural communities, and an overall reduction in microbial diversity and stability in western populations [4] , [9] . Unindustrialized small-scale rural societies are targets for understanding trends in human–GM interactions because they rely less on antibiotics and sterile cleaners, and often consume a greater breadth of unrefined seasonally available foods [10] . Yet, despite recent focus on rural societies, there remains a significant gap in our knowledge of the microbe–host relationship among hunter-gatherer populations. This is especially problematic because humans have relied on hunting and gathering for 95% of our evolutionary history. Here, to explore how a foraging subsistence strategy influences GM profiles, we analyse faecal microbiota from 27 Hadza hunter-gatherers from two separate camp sites ( Fig. 1 ). The Hadza who chose to participate in this study came from the Dedauko and Sengele camps, situated in the Rift Valley ecosystem around the shores of Lake Eyasi in northwestern Tanzania. These participants are part of the ~200–300 traditionally living Hadza, who are one of the last remaining hunting and gathering communities in the world. The Hadza live in small mobile camps with fluid membership, usually comprising a core group of ~30 people, and target native wild foods, both hunted and foraged, for the bulk of their subsistence [11] . While the Hadza are a modern human population, they live in a key geographic region for studies of human evolution and target resources similar to those exploited by our hominin ancestors. The Hadza lifestyle therefore is thought to most closely resemble that of Paleolithic humans. 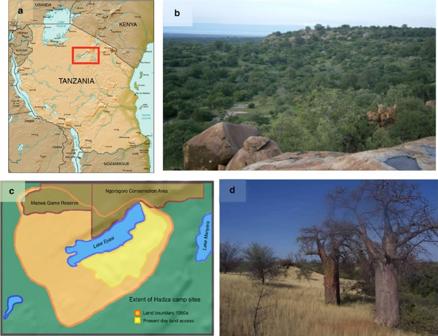Figure 1: Location and scenery of Hadza land in Tanzania, Africa. In deep bush camps, hunting and gathering still make up the majority (>90%) of subsistence. (a) Location of Hadza land in northern Tanzania; (b) top of a rock ridge near Sengele camp overlooking a lush landscape in between two phases of the rainy season; (c) extent of the land surrounding Lake Eyasi where Hadza make their camp sites, orange border denotes land area in 1950s and area in yellow shows the reduced area Hadza occupy today; (d) view of baobab trees within Hadza land during the early dry season. Photoamodified from the CIA World Factbook. Photosbanddby SL Schnorr and AN Crittenden. Figure 1: Location and scenery of Hadza land in Tanzania, Africa. In deep bush camps, hunting and gathering still make up the majority (>90%) of subsistence. ( a ) Location of Hadza land in northern Tanzania; ( b ) top of a rock ridge near Sengele camp overlooking a lush landscape in between two phases of the rainy season; ( c ) extent of the land surrounding Lake Eyasi where Hadza make their camp sites, orange border denotes land area in 1950s and area in yellow shows the reduced area Hadza occupy today; ( d ) view of baobab trees within Hadza land during the early dry season. Photo a modified from the CIA World Factbook. Photos b and d by SL Schnorr and AN Crittenden. Full size image We compare phylogenetic diversity, taxonomic relative abundance and the short-chain fatty-acid (SCFA) profile of the Hadza microbiome with those of 16 urban living Italian adults from Bologna, Italy. We then compare these data with previously published data on two different rural African groups from Burkina Faso (BF) and Malawi [4] , [9] to identify GM features unique to the Hadza lifestyle. This study presents the first characterization of a forager GM through work with the Hadza hunter-gatherers, and will allow us to understand how the human microbiota aligns with a foraging lifestyle, one in which all human ancestors participated before the Neolithic transition. Dietary information for sampled cohorts The Hadza diet consists of wild foods that fall into five main categories: meat, honey, baobab, berries and tubers ( Supplementary Table 1 and Supplementary Fig. 1 ) [12] , [13] , [14] . They practice no cultivation or domestication of plants and animals and receive minimal amounts of agricultural products (<5% of calories) from external sources [15] . 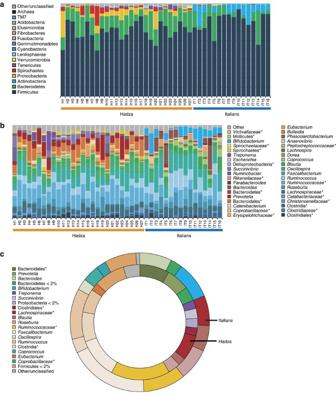Figure 2: Bacterial relative abundance of Hadza and Italian subjects. 16S rDNA gene survey of the faecal microbiota of 27 Hadza (H1-H27) and 16 Italian (IT1-IT16) adults. Relative abundance of (a) phylum and (b) genus-classified faecal microbiota is reported. Histograms are based on the proportion of OTUs per subject. Colours were assigned for all phyla detected, and for genera with a relative abundance ≥1% in at least 10% of subjects. (c) Donut charts summarizing genera relative abundance for Italians (outer donut) and Hadza (inner donut). Genera were filtered for those with ≥2% of total abundance in at least 10% of subjects. *denotes unclassified OTU reported at higher taxonomic level. By comparison, the diet of the Italian cohort derives almost entirely from commercial agricultural products and adheres largely to the Mediterranean diet: abundant plant foods, fresh fruit, pasta, bread and olive oil; low-to-moderate amounts of dairy, poultry, fish and red meat ( Supplementary Table 2 ). In addition, the majority of carbohydrates (based on gram amount) came from easily digestible starch (54%) and sugar (36%) while very little was derived from fibre-soluble or -insoluble (10%; Supplementary Fig. 2 ). 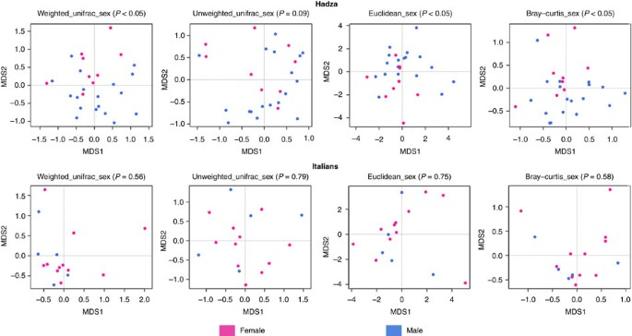Figure 3: Sex difference in GM structure among Hadza and Italians. PCoAs based on unweighted and weighted UniFrac distances as well as Euclidean and Bray–Curtis distances show patterns of separation by sex within each subject cohort and their respectiveP-values. Significance was calculated by permutation test with pseudoF-ratio. Pink, females; blue, males. Characterization of Hadza microbiota Faecal samples from 27 Hadza, aged 8–70 years, mean age 32 years and 16 Italians aged 20–40 years, mean age also 32 years ( Supplementary Table 3 ), were collected and pyrosequenced in the V4 gene region of bacterial 16S ribosomal DNA (rDNA), resulting in 309,952 high-quality reads and an average of 7,208±2,650 reads per subject. Reads were clustered into 11,967 operational taxonomic units (OTUs) at 97% identity. We used several different metrics to calculate α-diversity, including phylogenetic diversity [16] , OTU species count, the Chao1 index for microbial richness and the Shannon index for biodiversity ( Supplementary Fig. 3 ). Rarefaction curves for phylogenetic diversity plateaued after 4,000 reads per sample, approximating a saturation phase. All measures indicate a much higher GM diversity within the Hadza than in Italian samples ( P <0.001, the Mann–Whitney U -test). The Hadza and Italian samples show many notable differences in microbiota relative abundance, as a percent of reads assigned, at both phylum and genus levels ( Fig. 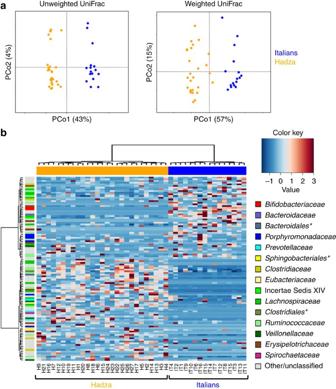Figure 4: GM phylogenetic difference between Hadza and Italian subjects. (a) Unweighted and weighted UniFrac distance PCoA of the faecal microbiota from 27 Hadza (orange dots) and 16 Italians (blue dots). (b) Hierarchical Ward-linkage clustering based on the Spearman correlation coefficients of genus proportion. Genera were filtered for subject prevalence of at least 30% within a population. Subjects are clustered on top of the panel and colour-coded as ina. Genera (110) clustered by the vertical tree are colour coded by family assignment. * denotes unclassified OTU reported at higher taxonomic level. 2 , Supplementary Table 4 ). In particular, the Hadza GM is largely dominated by Firmicutes (72±1.9%) and Bacteroidetes (17±1.1%). Other represented phyla are Proteobacteria (6±1.2%) and Spirochaetes (3±0.9%), with 2% of phylum level OTUs remaining unclassified. The most represented families in the Hadza GM are Ruminococcaceae (34%), Lachnospiraceae (10%), Prevotellaceae (6%) Clostridiales Incertae Sedis XIV (3%), Succinivibrionaceae (3%), Spirochetaceae (2%) and Eubacteriaceae (2%). Interestingly, a large number of taxa, the majority belonging to Bacteroidetes, Clostridiales, Bacteroidales and Lachnospiraceae , are unassigned at the level of family and genus, together representing 22% of the total community. Figure 2: Bacterial relative abundance of Hadza and Italian subjects. 16S rDNA gene survey of the faecal microbiota of 27 Hadza (H1-H27) and 16 Italian (IT1-IT16) adults. Relative abundance of ( a ) phylum and ( b ) genus-classified faecal microbiota is reported. Histograms are based on the proportion of OTUs per subject. Colours were assigned for all phyla detected, and for genera with a relative abundance ≥1% in at least 10% of subjects. ( c ) Donut charts summarizing genera relative abundance for Italians (outer donut) and Hadza (inner donut). Genera were filtered for those with ≥2% of total abundance in at least 10% of subjects. *denotes unclassified OTU reported at higher taxonomic level. Full size image To explore variation within the Hadza GM, we used weighted and unweighted UniFrac distances to assess differences based on camp location and sex. We found no significant difference in phylogenetic diversity or relative abundance between camps ( Supplementary Fig. 4 ). However, unlike the Italian cohort, the Hadza GM does show significant separation by sex based on weighted UniFrac distance ( P <0.05, permutation test with pseudo F -ratio). Analogous results were obtained when Euclidean and Bray–Curtis distance of genera relative abundance were considered ( P <0.05, permutation test with pseudo F -ratio; Fig. 3 ). To determine a structural basis for the observed separation, we compared genera relative abundance between Hadza men and women using a Mann–Whitney U -test, and found a significantly increased abundance of Treponema ( P <0.05) in women and increased Eubacterium ( P <0.05) and Blautia ( P <0.001) in men. These differences may result from the pronounced sexual division of labour and sex differences in diet composition among the Hadza [17] . Women selectively forage for tubers and plant foods, and spend a great deal of time in camp with children, family members and close friends. Men are highly mobile foragers and range far from the central camp site to obtain game meat and honey [18] . Although all foods are brought back to camp and shared, men and women consume slightly more of their targeted foods from snacking throughout the day [19] . The increased Treponema among women may be an adaptation to the higher amount of plant fibre in their diet, especially from tubers. Treponema is considered an opportunistic pathogen in industrialized populations because of T. pallidum , the bacterium responsible for syphilis and yaws [20] . However, this genus also includes proficient cellulose and xylan hydrolyzers [21] , and it is possible Treponema acts as a mutualistic component of the Hadza GM to help with fibre degradation. The sex-based divisions in the Hadza lifestyle probably play a role in altering composition abundance of the GM through different patterns of environmental and community exposure, such as those previously viewed across age, geography or diet [4] , [9] . Further clarification of this division would require the inclusion of more Hadza women in the sample pool. Figure 3: Sex difference in GM structure among Hadza and Italians. PCoAs based on unweighted and weighted UniFrac distances as well as Euclidean and Bray–Curtis distances show patterns of separation by sex within each subject cohort and their respective P -values. Significance was calculated by permutation test with pseudo F -ratio. Pink, females; blue, males. Full size image Detailed comparison with Italian controls The Hadza and Italian GM profiles are quite distinct. Community structure visualized using principal coordinates analysis (PCoA) of weighted and unweighted UniFrac distances reveal a sharp segregation along PCo1, indicating a strong core division in GM phylogeny between Hadza and Italian individuals ( P <0.001, permutation test with pseudo F -ratio; Fig. 4 ). Mean values of unweighted UniFrac distances also reveal lower within-group variability of taxonomic diversity among Hadza than Italians ( P <0.001, permutation test with pseudo F -ratio). This similarity in breadth of phylogenetic diversity among Hadza is probably a result of close proximity community living with food sharing. Camp movement is usually resource driven (food and water) and the size and duration of camps vary greatly by season. In the dry season, many groups congregate around water holes, which also make hunting more productive. During the wet season, groups are small and much more scattered with often five or fewer adults. Figure 4: GM phylogenetic difference between Hadza and Italian subjects. ( a ) Unweighted and weighted UniFrac distance PCoA of the faecal microbiota from 27 Hadza (orange dots) and 16 Italians (blue dots). ( b ) Hierarchical Ward-linkage clustering based on the Spearman correlation coefficients of genus proportion. Genera were filtered for subject prevalence of at least 30% within a population. Subjects are clustered on top of the panel and colour-coded as in a . Genera (110) clustered by the vertical tree are colour coded by family assignment. * denotes unclassified OTU reported at higher taxonomic level. Full size image Although Firmicutes and Bacteroidetes are the dominant phyla in both Hadza and Italian GM, Hadza are characterized by a relatively higher abundance of Bacteroidetes and a lower abundance of Firmicutes ( Supplementary Table 4 ). The two GM ecosystems are remarkably different with respect to subdominant phyla (<10% relative abundance). Hadza are largely enriched in Proteobacteria and Spirochaetes, which are extremely rare in the Italian GM, while Actinobacteria, an important subdominant component of the Italian GM, are almost completely absent from the Hadza microbiome. At the genus level, the Hadza GM is comparatively enriched in Prevotella , Eubacterium , Oscillibacter , Butyricicoccus , Sporobacter , Succinivibrio and Treponema and correspondingly depleted in Bifidobacterium , Bacteroides , Blautia , Dorea , unclassified Lachnospiraceae , Roseburia , Faecalibacterium , Ruminococcus and unclassified Erysipelotrichaceae . Moreover, there are many unclassified genera belonging to Bacteroidetes, Clostridiales and Ruminococcaceae in the Hadza GM, emphasizing our still limited ability to identify community-dependent bacteria. 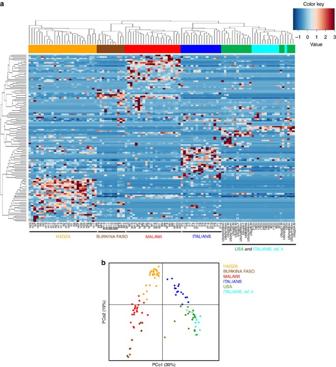Figure 5: Comparison of GM relative abundance among populations reflects subsistence patterns. (a) Hierarchical clustering based on Eisen’s formula of correlation similarity metric of bacterial genus proportion and average linkage clustering. Genera were filtered for subject prevalence of at least 30% of samples. Subjects are clustered in the top of panel and colour-coded orange (Hadza), brown (BF), red (Malawi), blue (Italian adult controls from this study), green (US adults from ref.9) and cyan (Italian children from ref.4). Genera (107) are visualized and clustered by the vertical tree. (b) PCoA based on Bray–Curtis distances of the relative abundance of GM genera of each population. The absence of Bifidobacterium in the Hadza GM was confirmed by quantitative PCR (qPCR; Supplementary Table 5 ). Taken together, data from our GM comparative analysis indicate a characteristic configuration for the Hadza gut microbial ecosystem that is profoundly depleted in Bifidobacterium , enriched in Bacteroidetes and Prevotella , and comprises an unusual arrangement of Clostridiales. This arrangement is defined by a general reduction of well-known butyrate producers, members of the Clostridium clusters IV and XIVa [22] and a corresponding increase in unclassified Clostridiales and Ruminococcaceae . Interestingly, the Hadza GM is also characterized by a relevant enrichment in what are generally considered opportunistic microorganisms, such as members of Proteobacteria, Succinivibrio and Treponema . Comparison with African agricultural societies The Hadza GM shares some features with other African populations, namely, enrichment in Prevotella, Succinivibrio and Treponema [4] , [9] , [23] . Therefore, to explore community-level relationships within the GM that may be unique to a foraging lifestyle, we sought associations among genera by including two previously published rural African groups with an agriculture-based subsistence and their respective western controls: 11 Mossi children from the Boulpon village, BF aged 5–6 years and 12 Italian children aged 3–6 years [4] ; 22 young adult members from four rural Malawian communities, Chamba, Makwhira, Mayaka and Mbiza aged 20–44 years and 17 US adults aged 24–40 years [9] . Clustering analysis shows a significant ( P <0.001, Fisher’s test) separation among Hadza, Malawians, BF and western controls ( Fig. 5a ). PCoA based on Bray–Curtis distances of genera relative abundance confirms this separation ( P <0.001, permutation test with pseudo F -ratio; Fig. 5b ). Interestingly, PC1, which represents the 30% of the total variability, shows a clear separation between the western controls and the African populations, while PC2, which explains a lower fraction of the total variability (19%), indicates a separation among Hadza, Malawians and BF. Separation along PC2 is also visualized among western populations, but to a much lesser degree and with large interspersion between the US and Italian children. Our data demonstrate biologically meaningful variation between the western and non-western GM profiles, showing that African populations with different lifestyles possess an overall more similar GM to each other than to western populations. Although these results indicate a certain degree of GM variation among different African groups, we cannot exclude that a study effect may outweigh separation owing to actual differences in GM composition within these communities. While we do see that the US controls intersperse with the Italian children (green and light blue colour coding, respectively), the Italian adults from this study remain distinct from the other western control samples, indicating that there may be some methodological bias that could also affect the observed GM differences among the African populations. Therefore, we urge caution in interpreting the strength of GM variation based on the separation seen among Hadza, BF and Malawian populations in this single cross-study comparison. Further caution is needed since subjects from all six populations are not age matched. Figure 5: Comparison of GM relative abundance among populations reflects subsistence patterns. ( a ) Hierarchical clustering based on Eisen’s formula of correlation similarity metric of bacterial genus proportion and average linkage clustering. Genera were filtered for subject prevalence of at least 30% of samples. Subjects are clustered in the top of panel and colour-coded orange (Hadza), brown (BF), red (Malawi), blue (Italian adult controls from this study), green (US adults from ref. 9 ) and cyan (Italian children from ref. 4 ). Genera (107) are visualized and clustered by the vertical tree. ( b ) PCoA based on Bray–Curtis distances of the relative abundance of GM genera of each population. Full size image To identify patterns of microbial community variation among Hadza, Malawian, BF and western controls—Italian adults, Italian children and US adults—we determined co-abundance associations between genera and then clustered them, resulting in six co-abundance groups (CAGs; Supplementary Fig. 5 ) [24] . In the context of this comparison, six CAGs define the microbial variation between populations ( P <0.001, permutational multivariate analysis of variance). CAGs have been named according to the dominant genera in each group as follows: Dialister , Faecalibacterium , Prevotella , Blautia , Clostridiales_ unclassified and Ruminococcaceae_ unclassified. The Wiggum [24] plot depicts the GM compositional relationship for each of the six populations and shows a correspondingly unique pattern of abundance of the six CAGs ( Fig. 6 ). Interestingly, African populations are characterized by the Prevotella CAG, while western controls show a distinctive overall dominance of the Faecalibacterium CAG. With respect to Malawian and BF, Hadza show a peculiar combined enrichment of Clostridiales _unclassified, Ruminococcaceae _unclassified and Blautia CAGs. Given the dietary and lifestyle distinctions of each population, the CAG distribution in Hadza, Malawians, BF and western controls could represent predictable GM community specificity to three different modes of subsistence: foraging, rural farming and industrial agriculture, respectively. The unique CAG distribution of Hadza with respect to the other groups corresponds to the higher abundance of Treponema and unclassified Bacteroidetes and Ruminococcaceae co-residents in the Hadza microbiome. All Hadza we sampled share this configuration; therefore, we must posit the possibility that these bacteria and their co-residents confer a structural and functional asset responding to the specific needs of the Hadza lifestyle. However, more forager and subsistence agriculture communities should be sampled to learn what aspects of subsistence drive microbe community assimilation and whether variability is a result of environment, host selection or both. 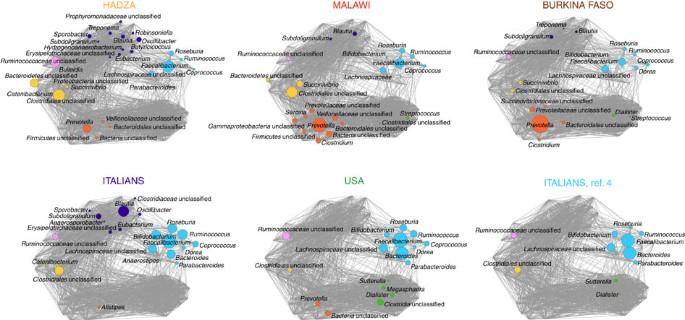Figure 6: Distinct bacterial co-abundance groups (CAGs) define each population. Wiggum plots indicate pattern of variation of the six identified CAGs in Hadza, Malawi, BF and western controls. CAGs are named with the name of the most abundant genera and are colour coded as follows:Faecalibacterium(cyan),Dialister(green),Prevotella(orange),Clostridiales_unclassified (yellow),Ruminococcaceae_unclassified (pink) andBlautia(violet). Each node represents a bacterial genus and its dimension is proportional to the mean relative abundance within the population. Connections between nodes represent positive and significant Kendall correlation between genera (FDR<0.05). Figure 6: Distinct bacterial co-abundance groups (CAGs) define each population. Wiggum plots indicate pattern of variation of the six identified CAGs in Hadza, Malawi, BF and western controls. CAGs are named with the name of the most abundant genera and are colour coded as follows: Faecalibacterium (cyan), Dialister (green), Prevotella (orange), Clostridiales _unclassified (yellow), Ruminococcaceae _unclassified (pink) and Blautia (violet). Each node represents a bacterial genus and its dimension is proportional to the mean relative abundance within the population. Connections between nodes represent positive and significant Kendall correlation between genera (FDR<0.05). Full size image SCFA profile of Hadza and Italians End products of bacterial fermentation are important for microbiota–host co-metabolism and evolution. SCFAs are the dominant metabolites resulting from bacterial fermentation of plant-derived substrates such as glycans and polysaccharides that pass undigested through the small intestine and into the colon. The SCFAs acetate, butyrate and propionate are pivotal in several host physiological aspects such as nutrient acquisition, immune function, cell signalling, proliferation control and pathogen protection [25] . Detected SCFA values for each sample are reported in Supplementary Table 6 . Principal component analysis of the SCFA relative abundance profiles shows a segregation between Hadza and Italians ( P =0.02, permutation test with pseudo F -ratio; Fig. 7 ). The Italian samples are characterized by a significantly ( P <0.01, the Mann–Whitney U -test) greater relative abundance of butyrate, while Hadza samples are enriched in propionate ( P <0.01, the Mann–Whitney U -test). These differences may reflect dietary variation in both amount and type of fibre and carbohydrates consumed by Hadza and Italians, and the consequent relative depletion in butyrate producers belonging to the Clostridium cluster IV and XIVa in Hadza. However, because of the high degree of metabolic cross-feeding between members of the human gut microbial ecosystem [26] , direct associative relations between bacteria presence/absence and SCFA production are not so simple. To investigate gut microbial networks on the basis of the observed differences in patterns of SCFA production in Hadza and Italians, we evaluated the GM genera that correlate significantly with each SCFA ( Supplementary Data 1–4 ). Among genera with greater than 5% relative abundance in at least one of the two populations, Bifidobacterium , Bacteroides , Blautia , Faecalibacterium and Ruminococcus are positively ( P <0.05, the Kendall tau rank-correlation coefficient) correlated with butyrate, showing the Kendall correlation values of 0.30, 0.31, 0.32, 0.52 and 0.30, respectively. In contrast, Bifidobacterium , Blautia and Lachnospiraceae show a significant ( P <0.05, the Kendall tau rank-correlation) negative correlation with propionate of −0.36, −0.27 and −0.24, respectively, while Prevotella demonstrates a positive correlation of 0.41. The absence of Bifidobacterium and the lower relative abundance of Blautia , Ruminococcus and Faecalibacterium concurrent with greater relative abundance of Prevotella seen in the Hadza GM match a presence/absence scenario with SCFA concentrations that are enriched in propionate and reduced in butyrate with respect to Italians. 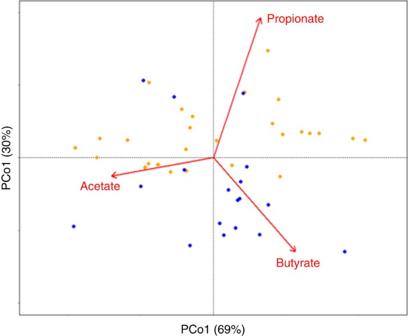Figure 7: Comparison of metabolite production between Hadza and Italian samples. PCoA based on Euclidean distances of the profiles of SCFA relative abundance in Hadza (orange) and Italians (blue). Vectors show propionate, butyrate and acetate abundance. Figure 7: Comparison of metabolite production between Hadza and Italian samples. PCoA based on Euclidean distances of the profiles of SCFA relative abundance in Hadza (orange) and Italians (blue). Vectors show propionate, butyrate and acetate abundance. Full size image Although SCFAs are metabolic end products for bacteria, they are important direct energy resources for the host. Butyrate is produced from dietary fibre, and when present in sufficient quantity, it becomes the major fuel source for colonic epithelial cells, reducing the need for energy allocation to these cells from the host [22] . Propionate is transferred to the liver where it serves as a precursor for hepatic gluconeogenesis [1] , [22] , [25] . The extra energy derived from these GM-produced SCFAs may provide nutritional support for the Hadza whose diet contains high amounts of fibre but is seasonally lean in lipids. The Hadza represent a rare example of human subsistence through hunting and gathering that persists in the same East African region where early hominins lived. The Hadza maintain a direct interface with the natural environment, deriving their food, water and shelter from a rich biosphere blanketed in the complexity of microbial communities and interactions. In our characterization of the Hadza GM, we report several findings that we feel support the conception of the microbiome as a diverse and responsive ecosystem adapting continuously as a commensal component of the host supra-organism. Keeping this framework in mind, we interpret the GM structure as an adaptation to the Hadza foraging lifestyle. The Hadza GM has characteristic features that are consistent with a heavily plant-based diet. Besides the presence of several well-known fibre-degrading Firmicutes that are also shared with Italians—for example, members of Lachnospiraceae , Ruminococcaceae , Veillonellaceae , Clostridiales Incertae Sedis XIV and Clostridiaceae , the Hadza GM is enriched in Prevotella, Treponema and unclassified members of Bacteroidetes, Clostridiales and Ruminococcaceae . These xylan-degrading Prevotella [26] and Treponema [21] and the abundance of still unclassified Bacteroidetes and Clostridiales, groups known for their fibrinolytic capabilities, may provide the Hadza GM with specific glycan-degrading abilities for Hadza to deal with a vast array of refractory and resistant organic materials that are introduced through diet. Consistent with GM arrangements reported for other African groups [4] , [9] , [23] , the Hadza GM shows a higher relative abundance of Prevotella , but with a correspondent reduction of Bacteroides in the gut ecosystem compared with the Italian control cohort. Thus, similar to what has been proposed for rural Africans consuming grain-based high-fibre diets [4] , it is tempting to speculate that this microbe community within the Bacteroidetes phylum could harbour the necessary GM functions for Hadza to deal with their especially unique, but also highly fibrous, plant food dietary constituents [27] . During our visit in January 2013, between two rainy periods, there were a variety of foods available and acquired, the majority of which were derived from plants. These included at least four species of tuber, small and large game, honey from stinging and stingless bees, leafy green foliage, baobab fruit and one species of berry ( Supplementary Table 1 ). Tubers are an incredibly important food in the Hadza diet because they are consistently available and exploited year round, despite being the lowest-ranked food resource [14] . Hadza tubers are uncultivated wild species belonging to the plant families Fabaceae (legumes), Convolvulaceae (morning glories and herbaceous vines) and Cucurbitaceae (squashes, melons and gourds). Only the underground root is harvested and consumed either raw or briefly roasted. It is noteworthy that most of the tubers consumed by Hadza contain high moisture and tough indigestible fibres that must be expectorated as a quid during chewing ( Supplementary Fig. 1 ). The digestible fraction is thus incredibly variable but composed of largely water, simple sugars, starch and soluble fibre. Several publications have outlined the basics of Hadza diet [12] , [13] , [15] , [28] , [29] , [30] and have converged on the following general characteristics. The majority of the annual Hadza diet (~70% of kilocalories) comes from plant foods [15] . Birds, small, medium and large-sized game meat comprise ~30% of the annual diet [15] . See refs 15 and 30 for an exhaustive list of all species targeted. Small variation exists between published sources depending on whether kilogram wet weight or kilocalories per gram were used to calculate percent contribution to diet. Resource availability—both plant and animal—is highly correlated with rainfall patterns; therefore, diet varies year to year as well as season to season. A general dietary pattern does emerge, however, and indicates that more meat is consumed during the dry season when people and game animals converge to target the same watering holes [31] . Foods like baobab, tubers and honey are targeted year round. On the basis of these data, the resulting picture is a diet rich in simple sugars, starch and protein while lean in fat. It would be of great interest to learn whether the shift from a largely plant-based diet to one that includes more meat, such as during the dry season, might show a concurrent change in GM structure amongst Hadza. We find evidence of a sex-related divergence in Hadza GM structure, which is not documented in other human groups. This divergence corresponds to the Hadza sexual division of labour and sex differences in diet composition. In the same environment with access to the same dietary resources, Hadza men and women are differentially adapted to their particular pattern of food consumption. The potential for Hadza women’s GM to respond with significant structural differences to the increased consumption of plant foods represents a profound break with traditional thinking on the limited digestive capacity of the human gut and the constraint it imposes on nutritional provisioning for reproduction and brain growth [32] , [33] . Women’s foraging must adequately provision for pregnancy and lactation, which is a strong adaptive pressure for the GM to derive the most energy from consistently available plant foods. In this regard, the GM aligns with the host nutrition acquisition strategy, thus potentially buffering women from resource ‘gaps’ that may lead to nutritional deficiencies. The reported presence of Treponema in now five geographically separate extant rural human communities from this and previous studies (Hadza, BF, Malawians, South Africans and Venezuelan Amerindians) [23] , [34] supports an alternative functional role for this bacterial group whose expression in industrialized communities is normally attributed to pathogenic disease. De Filippo et al. [4] hypothesize that the presence of Treponema in BF children enhance the host’s ability to extract nutrients from the fibrous foods that comprise their traditional diet. While the Hadza do not eat agricultural or grain-based diets, they do rely heavily on fibrous tubers throughout the year, with women often consuming tubers for a greater percentage of daily calories than do men [19] . These sources of fibre-rich plant foods could similarly encourage a mutualistic Treponema population whose fibrinolytic specializations would be advantageous to Hadza nutritional acquisition, particularly in women. Medical examinations conducted on Hadza found evidence of Treponematosis from serum samples at low rates (13 out of 215 sampled) with the highest prevalence in men of settled Hadza camps between 1966 and 1967 (ref. 35 ). However, there was low but consistent prevalence for women in both settled and foraging Hadza groups with little clinical evidence of yaws, suggesting immunoregulation of Treponema pathogens. Demographic reports of age structure, population density, growth and fertility indicate that the Hadza appear to be a healthy and stable savanna foraging population despite rapid encroachment of pastoralist groups in the same region [11] . For a foraging population with little to no access to healthcare or medical facilities, the Hadza have relatively low rates of infectious disease, metabolic disease and nutritional deficiencies in comparison with other settled groups in the northern Tanzania and southeastern Uganda region [11] , [35] , [36] . However, these earlier assessments were more than 40 years ago, over two Hadza-generations, and many changes have since occurred to the land occupied by the Hadza. Re-evaluation of health and population metrics deserves renewed focus, especially now that research on the Hadza has garnered much attention. The absence of Actinobacteria, particularly Bifidobacterium , in the Hadza GM is unexpected. Bifidobacteria are associated with breastfeeding in infants and achieve large proportions of the GM in the first few months after birth [37] . Typically, in adults, bifidobacteria commonly make up 1–10% of the GM population. Complete absence of bifidobacteria, as observed in the Hadza, has never to our knowledge been reported for any other human group. We hypothesize that the lack of bifidobacteria in adult Hadza is a consequence of the post-weaning GM composition in the absence of agro-pastoral-derived foods. Support for this hypothesis comes from the observation that other populations in which meat and/or dairy consumption is low to absent, such as vegans and Koreans, also have very low representation of Actinobacteria and Bifidobacterium [38] , [39] . The continued consumption of dairy into adulthood could be one reason most western populations maintain a relatively large bifidobacterial presence. Aside from bifidobacterial species of human origin, the majority of Bifidobacterium have been isolated from livestock animals such as swine, cattle and rabbit [37] , [40] . The Hadza neither domesticate nor have direct contact with livestock animals. Thus, as they lack exposure to livestock bifidobacteria, this raises the question of whether the necessary conditions for interspecies transfer and colonization of bifidobacteria do not occur for the Hadza [41] . The Hadza retain a strong independent identity both in their native language and oral history, which says nothing about a previous pastoral or agricultural existence [15] . Early Y chromosome and mitochondrial DNA analysis shows some of the highest genetic divergence between Hadza and members of the Khoisan/San language group, the Ju/’hoansi (!Kung), evidence suggestive of a very ancient lineage [42] . Given their penchant for social timidity during early attempts at first contact and resistance to assimilation in the second half of the twentieth century, it is very likely the Hadza persist with a very ancient traditional lifestyle into present times [15] . Future work must focus on the GM of breast-fed Hadza infants to determine the role of bifidobacteria in the kinetics of assembly and development of the Hadza GM, and to learn whether this bacterial group is completely absent in all Hadza, including infants, or whether it is definitively lost from the gut ecosystem post weaning. It is important to note that while bifidobacteria are considered a beneficial bacterial group in western GM profiles, their absence in the Hadza GM, combined with the alternative enrichment in ‘opportunistic’ bacteria from Proteobacteria and Spirochaetes, cannot be considered aberrant. On the contrary, the Hadza GM probably represents a new equilibrium that is beneficial and symbiotic to the Hadza living environment. Support for the advantage of such novel GM configurations comes from the finding that GM restructuring also occurs in centenarians [43] , who are extreme examples of organismal robusticity. In addition, these findings illustrate a need to reevaluate the standards by which we consider GM ‘healthy’ or ‘unhealthy’, as they are clearly context dependent. GM diversity, as found in rural African populations and now in the Hadza, is almost certainly the ancestral state for humans. Adaptation to the post-industrialized western lifestyle is coincident with a reduction in GM diversity, and as a result, a decline in GM stability. Diversity and stability are factors with major health implications, particularly now that the human gastrointestinal tract is increasingly recognized as the gateway to pathogenic, metabolic and immunologic diseases [44] . Co-speciation between host and microbiota over millions of years has shaped both sets of organisms into mutualistic supra-organisms. Dissolving that contact through sterilization and limited environmental exposure has had a drastic effect on health and immune function of modern westernized human groups. The Hadza GM is likely an ‘old friend’ and stable arrangement fitting their traditional hunter-gatherer lifestyle [45] . We are only just beginning to document GM diversity across populations. In our study, more than 33% of the total Hadza GM genera remain unidentified. Such taxonomic uncertainty holds exciting prospects for discovering yet unknown microbial genetic arrangements. This finding also underscores the importance of increasing our reference phylogenies and resolving deep taxonomic relationships between bacteria by sampling a wider variety of environments and extreme ecological zones [7] . In summary, the characterization of the Hadza GM presents a suite of unique features that suggest specific adaptation to a foraging lifestyle, which includes a large proportion of highly refractory plant foods. We expect that detailed study of the function of this GM community will expose a greater number of genetic specializations for degrading polysaccharides than what is currently found in other human populations. When viewed broadly, inconsistencies in associations among GM structure, diet and disease belie interpretive confidence about GM phenotypes. The functional redundancy found in bacterial communities indicates that microbial activity, rather than composition, is conserved. However, the ability of novel genes to propagate through environmental transfer into common gut bacteria complicates the enterotype–function paradigm. Moreover, closely related human symbiont microorganisms have been demonstrated to differ widely in their glycan use phenotypes and corresponding genomic structures [46] . Even if taxonomic similarities do exist between human populations, at finer scales their GM communities may exhibit dramatic metabolic differences tailored to suit disparate environmental constraints. With a microbiome functional assignment rate at 60% (ref. 2 ), these questions need to be resolved by testing GM activity using in vivo techniques such as with gnotobiotic mice [47] or in vitro techniques such as with computer-controlled simulations of the large intestine [48] . Furthermore, comparative analysis between the human and great ape GM, especially with members of Pan , will highlight important distinctions that enabled early human ancestors to extend their dietary and ecological ranges without the need for technological buffering. Host–microbiome mutualism holds great relevance to the field of human evolution as it vastly propels the genetic landscape for adaptation well beyond somatic potential. Subject enrollment The 27 Hadza volunteers who participated in this study came from the Dedauko and Sengele camps and are part of the ~200–300 traditionally living Hadza. Faecal samples were collected over a period of 2 weeks in January 2013 from consenting healthy participants. All participants were first told of the study, its objectives and their role as volunteers. Since Hadza are non-literate, verbal consent was obtained by those who agreed to participate, and this was documented by a separate witness. In the case of young Hadza, we obtained verbal assent from the youths and verbal consent from the parents, which was again documented by a separate witness. Samples were matched with subject interviews to record age, sex and health status, but because of ambiguity with regard to age of some of the participants, this information was excluded from further analysis. All work was approved by the University of Leipzig Ethik-Kommission review board on 29 May 2012, reference number 164-12-21052012. Permission for this work was granted from the Tanzanian Commission for Science and Technology (COSTECH), permit number 2012-315-NA-2000-80. Sixteen Italian adults (age: 20–40 years) were recruited for this study in the greater Bologna metropolitan area. All subjects were healthy and had not received antibiotics, probiotics or prebiotics for at least 3 months before sampling. Written informed consent was obtained from the subjects enrolled. Samples were collected between March and April 2013. Twenty-four hour dietary recalls were provided by each enrolled subject for 3 days. We used the standard method in nutritional science of sampling 2 week days and 1 weekend day in an attempt to fully account for dietary habit and fluctuation. Records were entered and analysed using the Food Processor SQL version 10.13.0 and compiled for summary reporting of the main caloric contributions by food group and macronutrient. Sample collection and storage Hadza samples were handled and stored following previously described methods [49] . In brief, samples were submerged in 30 ml of 97% ethanol for 24–36 h, after which the ethanol was carefully poured out and the remaining solid material was transferred to 50 ml tubes containing silica beads (Sigma 10087). All Hadza samples were transported by express to Bologna, Italy where further analysis was performed. Italian samples were collected, dried using the two-step ethanol and silica procedure, and stored at −80 °C in Bologna until further use. Comparison of dry and frozen faecal samples Hadza stool samples could not remain frozen during their removal from Tanzania because of unreliable sourcing of dry ice shipping materials, so we first performed a comparison of DNA extraction and amplification and SCFA quantification on split samples of Germany-living westerners. Stool samples were split into two segments, one fraction was stored at −80 °C and the second was dried using the two-step ethanol/silica procedure as described above. Total DNA extraction yield, pyrosequencing of the 16S rDNA V4 gene region and SCFA relative abundance quantification were performed (as described below) in parallel from frozen and dried sample aliquots. According to our data, we obtained comparable DNA yield, GM profiles and SCFA relative abundance profiles from frozen and dry aliquots of the same stool ( Supplementary Table 7 ). GM profiles were shown to cluster by subject independent of the storage method ( Supplementary Fig. 6 ). Taken together, these data support the reliability of the drying method for use in stool storage. DNA extraction from faecal samples Total DNA from faecal material was extracted using QIAamp DNA Stool Mini Kit (QIAGEN) with a modified protocol. In brief, 250 mg of faeces were suspended in 1 ml of lysis buffer (500 mM NaCl, 50 mM Tris–HCl pH 8, 50 mM EDTA, 4% SDS). Four 3 mm glass beads and 0.5 g of 0.1 mm zirconia beads (BioSpec Products) were added, and the samples were treated in FastPrep (MP Biomedicals) at 5.5 movements per second for 3 min. Samples were heated at 95 °C for 15 min, and then centrifuged for 5 min at full speed to pellet stool particles. Supernatants were collected and 260 μl of 10 M ammonium acetate was added, followed by incubation in ice for 5 min and centrifugation at full speed for 10 min. One volume of isopropanol was added to each supernatant and incubated in ice for 30 min. The precipitated nucleic acids were collected by centrifugation for 15 min at full speed and washed with ethanol 70%. Pellets were resuspended in 100 μl of TE buffer and treated with 2 μl of DNase-free RNase (10 mg ml −1 ) at 37 °C for 15 min. Protein removal by Proteinase K treatment and DNA purification with QIAamp Mini Spin columns were performed following the kit protocol. Final DNA concentration was determined by using NanoDrop ND-1000 (NanoDrop Technologies). 16S rDNA gene amplification For the amplification of the V4 region of the 16S rDNA gene, the primer set 520F (5′-AYTGGGYDTAAAGNG-3′) and 802R (5′-TACNVGGGTATCTAATCC-3′) (with Y=C/T, D=A/G/T, N=any base, V=A/C/G) was used. These primers were designed to include at their 5′-end one of the two adaptor sequences used in the 454-sequencing library preparation protocol (adaptor A and B), linked to a unique MID tag barcode of 10 bases allowing the identification of the different samples. PCR mixtures contained 0.5 μM of each forward and reverse primer, 100 ng of template DNA, 2.5 U of GoTaq Flexi Polymerase (Promega), 200 μM of dNTPs and 2 mM of MgCl 2 in a final volume of 50 μl. Thermal cycling consisted of an initial denaturation step at 95 °C for 5 min, followed by 35 cycles of denaturation at 94 °C for 50 s, annealing at 40 °C for 30 s and extension at 72 °C for 60 s, with a final extension step at 72 °C for 5 min (ref. 50 ). PCR amplifications were carried out in a Biometra Thermal Cycler T Gradient (Biometra). qPCR for Bifidobacterium quantification qPCR was carried out in a LightCycler instrument (Roche). Quantification of the 16S rRNA gene of Bifidobacterium was performed with previously described genus-specific primers bif-164 and bif-662 (ref. 51 ). For quantification, standard curves were generated by using 10-fold serial dilution of genomic DNA from B. animalis subspecies lactis BI07. Amplification was carried out in a 20-μl final volume containing 100 ng of faecal DNA, 0.5 μM of each primer and 4 μl of LightCycler-FastStart DNA Master SYBR Green I (Roche). Amplifications were done under the following conditions: (i) starting preincubation at 95 °C for 10 min; (ii) amplification including 35 cycles of four steps each at the temperature transition rate of 20 °C s −1 : denaturation at 95 °C for 15 s, annealing at 63 °C for 20 s, extension at 72 °C for 30 s and fluorescence acquisition at 90 °C for 5 s; and (iii) melting curve analysis. Pyrosequencing of faecal slurries The PCR products derived from amplification of the specific 16S rDNA V4 hypervariable region were individually purified with MinElute PCR Purification Kit (QIAGEN) and then quantified using the Quant-iT PicoGreen dsDNA kit (Invitrogen). After the individual quantification step, amplicons were pooled in equal amounts (thus, creating three 9-plex for Hadza samples and two 8-plex pools for Italian samples) and again purified by 454-Roche Double Ampure size selection protocol with Agencourt AMPure XP DNA purification beads (Beckman Coulter Genomics GmbH) to remove primer dimers, according to the manufacturer’s instructions (454 LifeSciences, Roche). Amplicon pools were fixed to microbeads to be clonally amplified by performing an emulsion PCR following the GS-FLX protocol Titanium emPCR LIB-A (454 LifeSciences, Roche). Following this amplification step, the beads were enriched to keep only those carrying identical PCR products on their surface, and then loaded onto a picotiter plate for pyrosequencing reactions, according to the GS-FLX Titanium sequencing protocol. All pools were sequenced in one-eighth of a plate each. Bioinformatic analysis of 16S rDNA and statistical methods Sequencing reads were analysed using the QIIME pipeline [52] as described previously [24] . In brief, V4 sequences were filtered according to the following criteria: (i) read length not shorter than 150 bp and not longer than 350 bp; (ii) no ambiguous bases (Ns); (iii) a minimum average quality score over a 50-bp rolling window of 25; and (iv) exact match to primer sequences and maximum 1 error in barcode tags. For bacterial taxonomy assignment, we used RDP-classifier (version 2.2) with 50% as confidence value threshold. Trimmed reads were clustered into OTUs at 97% identity level and further filtered for chimeric sequences using ChimeraSlayer ( http://www.microbiomeutil.sourceforge.net/#A_CS ). Alpha-diversity and rarefaction plots were computed using four different metrics: Shannon, PD whole tree, chao1 and observed species. Weighted and unweighted UniFrac distances and Euclidean distance of genus-level relative abundance were used to perform PCoA. PCoA, heatmap and bar plots were built using the packages Made4 (ref. 53 ) and Vegan ( http://www.cran.r-project.org/package=vegan ). The R packages Stats and Vegan were used to perform statistical analysis. In particular, to compare GM structure among different populations for α and β diversity, we used a Wilcoxon-signed rank test. Data separation in the PCoA was tested using a permutation test with pseudo F -ratios (function Adonis in the Vegan package). Cluster separation in hierarchical clustering analyses was assessed for significance using Fisher’s exact test. Significant differences in phylum or genus-level abundance between Hadza and Italians, and between Hadza males and females, were assessed by Mann–Whitney U -tests, and corrected for multiple comparisons using the Benjamini–Hochberg method when appropriate. False discovery rate (FDR)<0.05 was considered as statistically significant. The Kendall correlation test between SCFA levels and the relative abundance of genera was achieved using function ‘cor.test’ of the package ‘Stats’ of R. Sequences from refs 9 and 4 and were obtained from Metagenomics Rapid Annotation using Subsystem Technology (MG-RAST), project I.D. 201 and European Nucleotide Archive, project number ERP000133, repositories, respectively, and processed and assigned following the QIIME pipeline. Bacterial CAGs were determined as described previously [24] . In brief, the associations among the genera were evaluated using the Kendall correlation test, visualized using hierarchical Ward clustering with a Spearman correlation distance metrics and used to define co-abundant genera groups. The significant associations were controlled for multiple testing using the q -value method (FDR<0.05) [54] . Permutational multivariate analysis of variance [55] was used to determine whether the CAGs were significantly different from each other. The Wiggum plot network analysis was created as previously described [24] using cytoscape software ( http://www.cytoscape.org/ ). Circle size represents genus abundance and connections between nodes represent positive and significant Kendall correlations between genera (FDR<0.05). GC–MS determination of SCFAs in faecal samples Aliquots of dried faecal samples (about 250 mg) were briefly homogenized after the addition of 1 ml of 10% perchloric acid in water and centrifuged at 15,000 g for 5 min at 4 °C. Five hundred microlitres of supernatant was diluted 1:10 in water, 10 μl of D8-butyric acid (internal standard, IS) were added to the sample at the final concentration of 20 μg ml −1 . The calibration curves were prepared adding the IS to scalar amounts of the acids in diluted samples or water (for external standardization). All the standards (purity >99%), acetic, propionic, butyric, valeric acids and IS were provided by Sigma and were used to prepare calibration solutions for quantification (linear response) and identification. Headspace solid-phase microextraction (HS-SPME) was performed by using a 75-μm Carboxen/polydimethylsiloxane fibre (Supelco). The optimized final extraction conditions were temperature 70 °C, 10 min of equilibration time and 30 min of extraction time. The analytes were desorbed into the gas chromatograph (GC) injector port at 250 °C for 10 min, including fibre cleaning. GC–mass spectrometry (MS) analysis was carried out on a TRACE GC 2000 Series (ThermoQuest CE Instruments) GC, interfaced with GCQ Plus (ThermoQuest CE Instruments) mass detector with ion trap analyser, operating in EI mode (70 eV). The capillary GC column was a Phenomenex ZB-WAX (30 m × 0.25 mm ID, 0.15 μm film thickness), consisting of 100% polyethylene glycol. Helium (He) was the carrier gas at a flow rate of 1.0 ml min −1 . An oven temperature programme was adopted: initial 40 °C (hold time: 5 min), then ramped by 10 °C min −1 to 220 °C (hold time: 5 min). The temperature of transfer line and ionization source was maintained at 250 and 200 °C, respectively. The GC was operated in splitless mode; the injector base temperature was set at 250 °C. The mass spectra were recorded in full scan mode (34–200 a.m.u.) to collect the total ion current chromatograms. Quantification was carried out by using the extracted ion chromatograms by selecting fragment ions of the studied analytes (43 and 60 a.m.u. for acetic acid, 55 and 73 a.m.u. for propionic acid, 60 and 73 a.m.u. for butyric and valeric acids, and 63 and 77 a.m.u. for IS). The SCFAs concentration in faecal samples was expressed in μmol g −1 of faeces. Limit of detection ranged from 4 to 68 nmol g −1 . Accession codes: Amplicon sequences have been deposited in the MG-RAST database under project ID 7058. How to cite this article: Schnorr, S. L. et al. Gut microbiome of the Hadza hunter-gatherers. Nat. Commun. 5:3654 doi: 10.1038/ncomms4654 (2014).